Genome evolution predicts genetic interactions in protein complexes and reveals cancer drug targets Genetic interactions reveal insights into cellular function and can be used to identify drug targets. Here we construct a new model to predict negative genetic interactions in protein complexes by exploiting the evolutionary history of genes in parallel converging pathways in metabolism. We evaluate our model with protein complexes of Saccharomyces cerevisiae and show that the predicted protein pairs more frequently have a negative genetic interaction than random proteins from the same complex. Furthermore, we apply our model to human protein complexes to predict novel cancer drug targets, and identify 20 candidate targets with empirical support and 10 novel targets amenable to further experimental validation. Our study illustrates that negative genetic interactions can be predicted by systematically exploring genome evolution, and that this is useful to identify novel anti-cancer drug targets. Knowledge of how proteins interact with each other to exert their function is crucial for understanding how disruption of interactions can lead to disease [1] , [2] and in the development of treatments. In recent years, several system-level maps of protein complexes have been constructed from physical interaction data [3] , [4] , [5] to initialize understanding of the functional relationships between proteins. These studies are important in identifying which proteins are linked to each other in biological processes [6] . Yet, these maps do not directly reveal how the proteins interact with each other. More specifically, they do not provide information about whether the interaction between two proteins is symmetric, in which both proteins are equally important in the function of a protein complex, or whether the interaction is asymmetric, in which one protein can function in the absence of the other protein, but not vice versa ( Fig. 1a ). One example of such asymmetry is the cyclin–Cdc28 complex where the function of the cyclin, Cln1p, depends on the Cdc28 kinase, but not vice versa . The function of Cln1p depends on Cdc28p as transcriptional activation of CLN1 requires an active Cdc28 kinase [7] . The function of Cdc28p, however, does not depend on Cln1p as the presence of Cln2p compensates for Cln1p’s absence to activate Cdc28p [8] (ref. 8 ). Thus, there is a functional asymmetry between Cln1p and Cdc28p, where Cln1p depends on Cdc28p and not vice versa (Cln1p→Cdc28p). Similarly, there is asymmetry between Cln2p and Cdc28p (Cln2p→Cdc28p). This example shows the relationship between functional asymmetry and what is called a negative genetic interaction, where mutations (for example, knockout) of two genes (for example, CLN1 and CLN2 ) reduce the fitness much more strongly than would be expected based on the decline in fitness of each gene individually [9] . The concept of negative genetic interactions is very valuable in the development of therapeutic treatments for diseases that can be treated by selectively depleting cells with a disease-causing mutation. Especially promising are the discoveries of cancer drugs that target proteins having synthetic lethal interactions with mutated oncogenes or tumour-suppressor genes [10] , [11] . The mechanism underlying this treatment is that inhibiting these genes separately is relatively harmless in a normal cell, while it is lethal to a cancer cell as it causes a lethal double mutant with mutated oncogenes/tumour-suppressor genes. Thus, targeting these genes can kill the cancer cells while leaving the normal cells relatively unaffected. Prioritizing drug targets in such an approach, by predicting negative genetic interactions between the mutated oncogenes/tumour-suppressor genes and other proteins, is, however, not trivial. 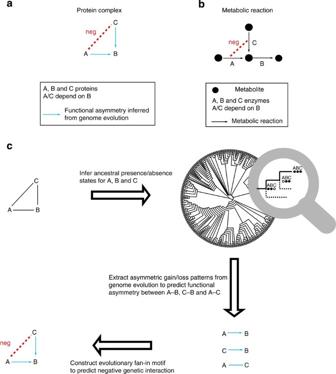Figure 1: Functional asymmetry and negative genetic interactions are linked. (a) Protein A and B have an asymmetric functional relationship, where the function of A depends on B but notvice versa. The asymmetry between protein A and B can be owing to the presence of protein C, which can compensate for a mutant of A. In such a scenario, proteins A and C are predicted to have a negative genetic interaction. (b) Functional asymmetry between enzyme A and B involved in a branched pathway in a metabolic network (A depends on B, but notvice versa: A→B). Nodes and arrows represent metabolites and reactions, respectively. The asymmetric relationship is owing to a converging reaction catalysed by enzyme C, which can compensate for A’s absence. Thus, enzyme A and C are likely to have a negative genetic interaction. (c) Flowchart to predict negative genetic interactions from genome evolution within a three-member protein complex (protein A, B and C). The blue arrow represents the functional asymmetry between two genes inferred from genome evolution. The blue line represents that there is no evolutionary evidence for a functional asymmetry between two genes. Here, both gene A and C are predicted to have functional asymmetry with B, while gene A and C are predicted not to have functional asymmetry. Figure 1: Functional asymmetry and negative genetic interactions are linked. ( a ) Protein A and B have an asymmetric functional relationship, where the function of A depends on B but not vice versa . The asymmetry between protein A and B can be owing to the presence of protein C, which can compensate for a mutant of A. In such a scenario, proteins A and C are predicted to have a negative genetic interaction. ( b ) Functional asymmetry between enzyme A and B involved in a branched pathway in a metabolic network (A depends on B, but not vice versa : A→B). Nodes and arrows represent metabolites and reactions, respectively. The asymmetric relationship is owing to a converging reaction catalysed by enzyme C, which can compensate for A’s absence. Thus, enzyme A and C are likely to have a negative genetic interaction. ( c ) Flowchart to predict negative genetic interactions from genome evolution within a three-member protein complex (protein A, B and C). The blue arrow represents the functional asymmetry between two genes inferred from genome evolution. The blue line represents that there is no evolutionary evidence for a functional asymmetry between two genes. Here, both gene A and C are predicted to have functional asymmetry with B, while gene A and C are predicted not to have functional asymmetry. Full size image Discovering negative genetic interactions mainly depends on laborious and specific experiments, which can be expensive and time-consuming, partially because of the explosion of the number of pairwise gene combinations. Several computational approaches have been developed to predict genetic interactions by integrating multiple types of functional genomic data, such as synthetic lethality data, physical interaction data and co-expression data [12] , [13] . These approaches, however, strongly depend on species-specific empirical genetic interaction data as input and therefore do not allow predictions for other species where genetic interaction data are largely unavailable. Here, we aim to predict negative genetic interactions in protein complexes via the concept of functional asymmetry, which we infer from genome evolution. The example of the cyclin-Cdc28 complex showed that functional asymmetry and negative genetic interaction are linked. This linkage can also be illustrated by enzyme relationships in metabolism. Enzymes in converging pathways have asymmetric relationships with an enzyme in an outgoing pathway [14] , [15] ( Fig. 1b ). Consequently, the enzymes in converging pathways can have negative genetic interactions, as they can compensate for each other’s absence. Analogous to metabolism, we expect that two proteins in a complex with asymmetry to a third protein will have a negative genetic interaction ( Fig. 1a ). Importantly, the functional asymmetry between enzymes in metabolism is indeed reflected in genome evolution [15] , [16] . On the basis of these prior studies, we have developed an evolutionary model to predict asymmetric functional relationships and negative genetic interactions in protein complexes in S. cerevisiae [17] . Our model predicts that almost 75% of the protein complexes in S. cerevisiae contain functionally asymmetric protein pairs. By integrating the information of predicted asymmetry in protein complexes, we show an up to twofold increase in the predictive power for negative genetic interactions relative to randomly chosen protein pairs from a complex. Moreover, our results show a twofold increase in prediction precision compared with an alternative model [18] . After mapping negative genetic interaction predictions from yeast to human, as well as a direct application to human protein complexes, we predict 20 cancer drug targets with empirical support and 10 completely novel targets not yet experimentally examined. Our study shows that higher-order functional relationships can be predicted by systematically exploring genome evolution, thereby providing a framework to interpret protein complex function with broad application to medical genetics. Functional asymmetry occurs frequently in protein complexes In order to examine if patterns in genome evolution can be used to predict negative genetic interactions, we first predicted asymmetry between protein pairs (A–B) in protein complexes from evolutionary analysis. We constructed a model integrating 11 evolutionary variables from the reconstructed ancestral states on a phylogenetic tree of 373 species ( Fig. 2 and Methods). For instance, evolutionary asymmetry between proteins A and B is inferred from the occurrence of multiple evolutionary loss events where only one of the two genes was lost in the descendant while both genes were present in the ancestor. If A is more frequently lost than B, then A is expected to be functionally dependent on B (A→B, see Fig. 2a , scenario f 1 ). The model was trained on a set of functionally asymmetric enzyme pairs in the genome-scale metabolic network of S. cerevisiae [19] to predict the dependency between the two enzymes (see Methods for detail). Using a tenfold cross-validation, the model showed a correct classification rate of 64.4% and an area under the receiver operator characteristic curve of 0.7 (see Methods for details; Supplementary Fig. S1 ). It should be noted that the performance of the model becomes worse when using a simpler model with only single gain and loss events ( Supplementary Fig. S1 ). We next asked how frequently functional asymmetry occurs in empirically determined protein complexes from S. cerevisiae [17] . Our analysis predicts that 71% (6,145 out of 8,711) of the protein pairs in these protein complexes are functionally asymmetric. Furthermore, ~75% (307 out of 409) of the protein complexes are found to have at least one predicted functionally asymmetric protein pair ( Supplementary Fig. S2 ). 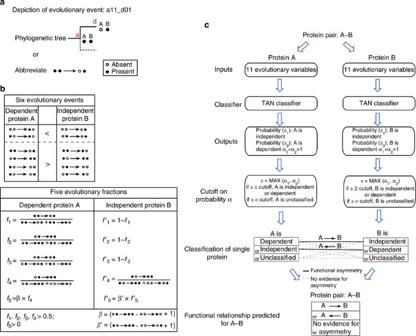Figure 2: Evolutionary variables to predict functional asymmetry. (a) Depiction of an evolutionary event. It shows a loss of gene A in the descendant (d) when both A and B are present in the ancestor (a). (b) Evolutionary variables used for the Bayesian classifier. The evolutionary variables across history of the dependent protein A in an asymmetric pair (A→B) can be expressed via 11 measures, listed in the first columns of two boxes. Of these 11, 6 count the number of times that a dependent protein A is gained or lost independently of B, including 2 that are expected to occur less often and 4 that are expected to occur more often for a dependent protein than for an independent protein. The remaining five measures are fractions that express relative frequencies of two evolutionary scenarios between A and B.f1,f2,f3andf4are expected to be larger than 0.5;f5, that weighsf4with the absolute difference between two gain events of A, is expected to be larger than 0. The six evolutionary and the five relative frequencies all contribute to the prediction of functional asymmetry (Supplementary Fig. S1). (c) Schematic presentation of predicting the functional asymmetry in a protein pair (A–B). A TAN classifier was trained on functionally asymmetric enzyme pairs in the metabolic network14. For a protein pair (A–B), the 11 evolutionary variables (Fig. 2b) are used to predict the conditional probability that A is functionally independent (α1) or dependent (α2). A is likely to be independent ifα1>α2, or dependent ifα1<α2. Subsequently, A can be predicted as independent, dependent or unclassified by applying a cutoff on probability (α=max(α1,α2), see Methods). The same procedure is applied to protein B. By combining the prediction of both, A–B can be either A→B where A is dependent and B is independent, B→A where A is independent and B is dependent, or no evidence for asymmetry when A and B have any other combination of predicted relationship. Figure 2: Evolutionary variables to predict functional asymmetry. ( a ) Depiction of an evolutionary event. It shows a loss of gene A in the descendant (d) when both A and B are present in the ancestor (a). ( b ) Evolutionary variables used for the Bayesian classifier. The evolutionary variables across history of the dependent protein A in an asymmetric pair (A→B) can be expressed via 11 measures, listed in the first columns of two boxes. Of these 11, 6 count the number of times that a dependent protein A is gained or lost independently of B, including 2 that are expected to occur less often and 4 that are expected to occur more often for a dependent protein than for an independent protein. The remaining five measures are fractions that express relative frequencies of two evolutionary scenarios between A and B. f 1 , f 2 , f 3 and f 4 are expected to be larger than 0.5; f 5 , that weighs f 4 with the absolute difference between two gain events of A, is expected to be larger than 0. The six evolutionary and the five relative frequencies all contribute to the prediction of functional asymmetry ( Supplementary Fig. S1 ). ( c ) Schematic presentation of predicting the functional asymmetry in a protein pair (A–B). A TAN classifier was trained on functionally asymmetric enzyme pairs in the metabolic network [14] . For a protein pair (A–B), the 11 evolutionary variables ( Fig. 2b ) are used to predict the conditional probability that A is functionally independent ( α 1 ) or dependent ( α 2 ). A is likely to be independent if α 1 > α 2 , or dependent if α 1 < α 2 . Subsequently, A can be predicted as independent, dependent or unclassified by applying a cutoff on probability ( α =max( α 1, α 2 ), see Methods). The same procedure is applied to protein B. By combining the prediction of both, A–B can be either A→B where A is dependent and B is independent, B→A where A is independent and B is dependent, or no evidence for asymmetry when A and B have any other combination of predicted relationship. Full size image Empirical evidence for functional asymmetry The high frequency of predicted functional asymmetry triggers the question to what extent our predictions are biologically meaningful. To answer this question, we asked whether predicted asymmetry is reflected in genome-scale empirical data. We first examined asymmetry in gene essentiality. For a predicted functionally asymmetric pair (A→B) where only one of the proteins is essential, we expect protein B to be the essential one. To test this, we examined those predicted asymmetric pairs where only one of the encoding proteins is essential and quantified to what extent the predicted asymmetry is consistent with asymmetry in gene essentiality. Our analysis reveals that 72% (1,071 out of 1,497) of the asymmetric pairs (A→B) are consistent with asymmetry in gene essentiality, that is, if one of the two genes is essential, it is B ( Fig. 3a ; one-tailed Fisher’s exact test; P <2.2e−16). 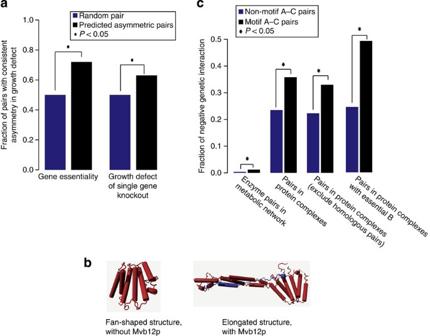Figure 3: Asymmetric functional relationships and negative genetic interactions. (a) Empirical support for predicted functional asymmetry in gene essentiality49and, for non-essential genes, in the growth defect of single-gene knockout20,21. For predicted asymmetric pairs (A→B), the fractionfAB(f01=n01/(n01+n10)), where 0=non-essential or no fitness defect and 1=essential or substantial growth defect is expected to be larger than 0.5 (fraction in pairs with no asymmetry). (b) One example of predicted functional asymmetry with experimental support. ESCRT-I is composed of four members, Vps23p, Vps28p, Vps37p and Mvb12p. Mvb12p (blue subunit) is predicted to functionally dependent on Vps23p, Vps28p and Vps37p (red) and notvice versa. Structural studies revealed that the functionally dependent subunit, Mvb12p, is a structural stabilizer, which changes the ESCRT-I core complex (Vps23p, Vps28p and Vps37p) from a fan-shaped structure (upper panel) to an elongated structure (lower panel)57. First, the dependency of Mvb12 on the core complex is supported by the fact that Mvb12p is unstable in cells lacking any of the other ESCRT-I subunits58. Second, that Vps23p, Vps29p and Vps37p do not strictly depend on Mvb12p is validated by the findings that certain MVB sorting pathways, such as carboxypeptidase S (CPS) and Ste2 sorting, are effective even if Mvb12p is absent58,59. However, loss of function of Vps23p, Vps28p or Vps37p results in a complete block of the MVB pathway58. (c) Enrichment of negative genetic interactions in fan-in motif A–C pairs. The fraction of negative genetic interaction is defined asf=Nneg/(Nneg+Npos+NnoInteraction).P-values in (a) and (c) were calculated with a one-tailed Fisher’s exact test and visualized with an asterisk (*) that stands for aP-value <0.05. Figure 3: Asymmetric functional relationships and negative genetic interactions. ( a ) Empirical support for predicted functional asymmetry in gene essentiality [49] and, for non-essential genes, in the growth defect of single-gene knockout [20] , [21] . For predicted asymmetric pairs (A→B), the fraction f AB ( f 01 = n 01 /( n 01 + n 10 )), where 0=non-essential or no fitness defect and 1=essential or substantial growth defect is expected to be larger than 0.5 (fraction in pairs with no asymmetry). ( b ) One example of predicted functional asymmetry with experimental support. ESCRT-I is composed of four members, Vps23p, Vps28p, Vps37p and Mvb12p. Mvb12p (blue subunit) is predicted to functionally dependent on Vps23p, Vps28p and Vps37p (red) and not vice versa . Structural studies revealed that the functionally dependent subunit, Mvb12p, is a structural stabilizer, which changes the ESCRT-I core complex (Vps23p, Vps28p and Vps37p) from a fan-shaped structure (upper panel) to an elongated structure (lower panel) [57] . First, the dependency of Mvb12 on the core complex is supported by the fact that Mvb12p is unstable in cells lacking any of the other ESCRT-I subunits [58] . Second, that Vps23p, Vps29p and Vps37p do not strictly depend on Mvb12p is validated by the findings that certain MVB sorting pathways, such as carboxypeptidase S (CPS) and Ste2 sorting, are effective even if Mvb12p is absent [58] , [59] . However, loss of function of Vps23p, Vps28p or Vps37p results in a complete block of the MVB pathway [58] . ( c ) Enrichment of negative genetic interactions in fan-in motif A–C pairs. The fraction of negative genetic interaction is defined as f = N neg /( N neg + N pos + N noInteraction ). P -values in ( a ) and ( c ) were calculated with a one-tailed Fisher’s exact test and visualized with an asterisk (*) that stands for a P -value <0.05. Full size image Many predicted asymmetric pairs have, however, no asymmetry in gene essentiality, simply because the majority of proteins are not strictly essential under standard laboratory conditions (that is, glucose-rich medium) [4] . Approximately 40% of the predicted asymmetric pairs are composed of two non-essential genes. Nevertheless, even when proteins are non-essential they can still contribute to fitness and result in significant growth defects after a gene knockout [20] , [21] . Similarly to the gene essentiality analysis, we expected that if one of the two proteins in a predicted asymmetric pair (A→B; both non-essential) has a stronger growth defect, it would be protein B. To test this, we examined 511 predicted asymmetric pairs where two non-essential proteins cause different growth defects, and quantified the consistency between the predicted and empirical functional asymmetry. As expected, 63% (322 out of 511) of the cases are consistent ( Fig. 3a ; one-tailed Fisher’s exact test; P =1.40e−04), that is, the predicted independent protein B has a stronger growth defect when knocked out. This consistency is robust at various cutoffs on empirical growth defect differences (ranging from 0.0001–0.3). Notably, the level of consistency increased from 63 to 67% when we increased the cutoff to 0.3, that is, where growth defect difference is largest. These results show that the evolutionary model is able to capture asymmetric functional relationships in protein complexes. ESCRT-I, a protein complex functioning in cargo selection in the multivesicular body (MVB) sorting pathway, is one example where the predicted functional asymmetry is supported by solid empirical evidence ( Fig. 3b ). Empirical evidence for negative genetic interactions An asymmetric functional relationship observed between two proteins A and B can also be linked to a type of relationship known as a negative genetic interaction [9] . The reasoning behind this is that B may not depend on the presence of A, because of the presence of another protein C that compensates for A’s absence. We asked whether our evolutionary model is capable of predicting such negative genetic interactions in multi-member protein complexes. We specifically focused on triplets where protein A, B and C are predicted to have an evolutionary fan-in motif ( Fig. 1a ). This motif is characterized by (i) A and C depend on B, but not vice versa and (ii) A does not depend on C and vice versa . This motif is analogous to converging pathways in metabolism, in which there is a mechanistic explanation for the compensatory effect between A and C ( Fig. 1b ). We therefore first investigated to what extent converging metabolic pathways [15] , [21] show negative genetic interactions [20] , [21] , [22] , [23] , [24] , [25] , [26] , [27] , [28] as a proxy for compensation, that is, double mutants cause more severe growth defects than expected from the two single mutants. Indeed, enzyme pairs in converging pathways show a threefold enrichment in negative genetic interactions compared with non-converging enzyme pairs ( Fig. 3c ; one-tailed Fisher’s exact test; P =2.42e−11). Given this result, we expect that in cases where we predict a fan-in motif within a protein complex, the A and C proteins have negative genetic interactions with each other. To address this, we compared fan-in A–C pairs with randomly chosen pairs from the same protein complex (that is, non-motif A–C pairs). Our results reveal that the fraction of negative genetic interactions increases by 50% when applying the evolutionary motif (from 23.5–35.8%; one-tailed Fisher’s exact test; P =0.00085; Fig. 3c ). It should be noted that this enrichment of negative genetic interactions is not owing to the functional complementation by homologous genes resulting from intra-complex gene duplications, as the results are hardly affected by removing homologous gene pairs (from 22.7–33.0%; one-tailed Fisher’s exact test; P =0.012; Fig. 3c ). As protein complexes are not necessarily active in standard laboratory conditions where genetic interactions have been measured, we expected that our test underestimates the predictive power. Indeed, when selecting for only protein complexes that are active in the cell (that is, B is essential) the predictive power even doubles (from 24.5–49.2%; one-tailed Fisher’s exact test; P =4.39e−05; Fig. 3c ). Thus, the evolutionary model can predict protein pairs that have a negative genetic interaction significantly and substantially more often than random pairs from protein complexes. To further assess the performance of our model, we compared the prediction precision and sensitivity of it with a model by Pandey et al. [18] by mapping their results to the protein complexes. This model has the highest known prediction accuracy and is also independent on genetic interaction information as input. Interestingly, our model has a twofold higher prediction precision (precision—TruePositives/TruePositives+FalsePositives: 0.36 versus 0.18; sensitivity—TruePositives/TruePositives+FalseNegatives: 0.47 versus 0.78). Notably, our model still has a precision of >0.3 when parameterized to the same sensitivity as Pandey’s model ( Supplementary Fig. S3 ). In total, our model predicted 273 A–C pairs in evolutionary fan-in motifs in S. cerevisiae protein complexes, for most of which (60%) a genetic interaction has not been measured. However, to provide empirical evidence for the predicted negative interactions, we exploited available genetic interaction data in Schizosaccharomyces pombe and Drosophila melanogaster via orthology definitions from STRING7.0 (ref. 29 ). Following this approach, we found that for ten out of our A–C pairs a genetic interaction has been experimentally found in either in S. pombe or in D. melanogaster and, as expected, most cases (8/10) show a negative genetic interaction in those species ( Supplementary Data 1 ). Negative genetic interactions reveal cancer drug targets The screen for negative genetic interactions has been shown to be a valuable strategy in the search for candidate cancer drug targets [10] , [30] . The common approach is to find proteins that have a negative genetic interaction with either an oncogene or a tumour-suppressor gene. As mutations in these genes cause cancer, the idea is that mutations in their negative genetic interaction partner would inhibit cancer cells to grow (that is, synthetic lethality) and leave normal cells relatively viable. Although a number of promising examples have been reported to target cancer cells via synthetic lethality [10] , [11] , [30] , discovering genetic interactions by experimental approaches is very labour intensive. Therefore, we asked whether our model captures conserved genetic interactions between S.cerevisiae and other species like D. melanogaster , such that it can serve as a framework to establish genetic interactions for medical genetics. Based on the orthologue profiles from STRING7.0 (ref. 29 ), we found 90.1% (246 out of 273) of the predicted fan-in motifs in yeast are conserved in D. melanogaster , that is, all three genes in a fan-in motif are present in D. melanogaster . Of these, nine have been examined for genetic interaction in D. melanogaster [31] , [32] , [33] , and all show negative genetic interaction (note, 7/9 have also been found in S.cerevisiae ). This suggests that our model can be used to predict negative genetic interactions in other species, such as mouse or human, which could provide a basis for prioritizing drug targets. To achieve the highest coverage, we combined two strategies to predict cancer drug targets: (i) by using orthology mapping from predicted negative interactions from yeast to human and (ii) by a direct application of our model to human protein complexes [34] , [35] . By using orthologues of the genes in the predicted fan-in motifs in yeast, we predicted ~250 novel negative genetic interaction pairs in human, of which 36 involve a cancer-related gene (oncogene or tumour-suppressor gene) [36] . Notably, most of these pairs (83.4%, 30/36) have not been reported before as negative genetic interactions. To apply our method directly on human protein complexes [34] , [35] , we first trained our model with functional asymmetric enzyme pairs from the human genome-scale metabolic network [37] (see Methods). Then we used the model to predict negative genetic interaction pairs. Totally, we predicted 1,012 gene pairs with negative genetic interactions of which 57 involve a cancer-related gene. Thus, totally, we predicted 93 cases with cancer-related genes. The genes that have a negative genetic interaction with these cancer-related genes are potential drug targets if they are essential in cancer cells while non-essential in normal cells. By examining gene essentiality in cancer cells [38] and non-essentiality in normal cells of Mus musculus (mouse), D. melanogaster or Danio rerio (zebrafish) ( Supplementary Data 2 ), we found that 30 out of the 93 involve promising cancer drug targets (pink column in Fig. 4 ; Supplementary Data 2 ). Among these 30 prioritized targets, 20 have been found to be essential in at least one cancer type, that is, breast, ovary or pancreas, and non-essential in a model organism (pink column in Fig. 4 ). Interestingly, most of these predicted targets (16/20) are essential in the exact cancer type where their negative genetic interaction partners, the cancer-related genes, are reported to be mutated or overexpressed (blue column in Fig. 4 ; Supplementary Data 2 ). This empirical evidence suggests that the lethality of the cancer cells by knockdown of the predicted target gene is actually caused by a lethal double mutant of the predicted targets and the cancer-related gene. As expected, when considering only those cases for which essentiality is measured in cancer cells (that is, 60+18 cases, green column in Fig. 4 ), the predicted targets are more likely to be essential in cancer and non-essential in normal cells compared with non-motif gene pairs (fraction E_cancer+NE_normal =0.26 versus 0.12, one-tailed Fisher’s exact test; P =4.8e−04). The remaining ten targets have not yet been experimentally examined for the essentiality in cancer cells: six are non-essential in M. musculus or D. melanogaster and four have not yet been measured (pink column in Fig. 4 ; Supplementary Data 2 ). Thus, we predicted 30 potential drug targets in total, that is, 20 with empirical support of essentiality in cancer cells and 10 novel ones ( Table 1 and Supplementary Data 2 ). To give an example, one of the predicted drug targets, TLE1 , has a negative genetic interaction with the cancer-related gene, HDAC1 (ref. 39 ). HDAC1 failed to be a direct drug target as the inhibition of mouse Hdac1 caused embryonic lethality in normal development [40] . TLE1 , on the other hand, has been found to be essential in several types of cancer cells [38] and non-essential in D. melanogaster [41] . In addition, TLE1 and HDAC1 have a confirmed negative genetic interaction in D. melanogaster [41] , which makes TLE1 a promising drug target for further analysis. 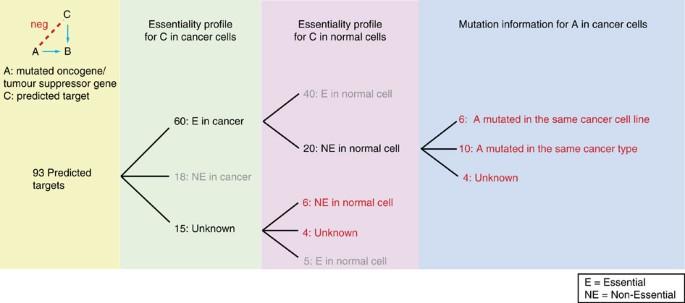Figure 4: Prioritized cancer drug targets with empirical support. Thirty prioritized cancer drug targets. The numbers in red represent the 30 promising targets. The numbers in grey represent the genes that failed to be targets as they are either non-essential in cancer cells or are essential in normal cells. In total, 93 genes are predicted to have a negative genetic interaction with a cancer-related gene. By examining gene essentiality in cancer and non-essentiality in normal cells, we prioritized 30 cancer drug targets. Twenty cases are essential in at least one cancer type, that is, breast, ovary or pancreas and non-essential in normal cells. Experimentally detected genetic variation/overexpression of the cancer-related gene and the RNA interference of the predicted targets in the same cancer type or the same cancer cell line were combined suggesting a double mutant. For most of these (16/20), there is empirical evidence that the cancer-related gene is mutated in either the same cancer type or the same cancer cell line as the predicted targets (blue column). For six cases that are confirmed to be non-essential in normal cells, the essentiality in cancer still needs to be examined experimentally. For four cases, the essentiality in both cancer cells and normal cells is not yet measured (red numbers in the pink column). Figure 4: Prioritized cancer drug targets with empirical support. Thirty prioritized cancer drug targets. The numbers in red represent the 30 promising targets. The numbers in grey represent the genes that failed to be targets as they are either non-essential in cancer cells or are essential in normal cells. In total, 93 genes are predicted to have a negative genetic interaction with a cancer-related gene. By examining gene essentiality in cancer and non-essentiality in normal cells, we prioritized 30 cancer drug targets. Twenty cases are essential in at least one cancer type, that is, breast, ovary or pancreas and non-essential in normal cells. Experimentally detected genetic variation/overexpression of the cancer-related gene and the RNA interference of the predicted targets in the same cancer type or the same cancer cell line were combined suggesting a double mutant. For most of these (16/20), there is empirical evidence that the cancer-related gene is mutated in either the same cancer type or the same cancer cell line as the predicted targets (blue column). For six cases that are confirmed to be non-essential in normal cells, the essentiality in cancer still needs to be examined experimentally. For four cases, the essentiality in both cancer cells and normal cells is not yet measured (red numbers in the pink column). Full size image Table 1 List of predicted cancer drug targets. Full size table Another example is the predicted interaction between NSUN2 and FBXW7 ( Fig. 5 ). NSUN2 is experimentally found to be essential in cancer cells [42] , and FBXW7 , a tumour-suppressor gene, has been found to be mutated in cancer cells [43] . In normal cells, NSUN2 and FBXW7 both function to regulate cellular differentiation via two different mechanisms. FBXW7 regulates cell differentiation by inhibiting c-Myc [44] and proteins in Notch pathway [45] , and NSUN2 functions to maintain normal cell differentiation when activated by LEF1/β-catenin complex, which is part of Wnt pathway [46] , [47] . It has been found that the loss of FBXW7 results in elevated expression of c-Myc [44] , which results in an upregulation of NSUN2 (ref. 48 ). As a result, NSUN2 stabilizes the mitotic spindle in fast cell proliferation in cancer cell growth [42] . Thus, targeting NSUN2 can kill cancer cells while leaving normal cells relatively unaffected, owing to the compensatory FBXW7–Notch pathway. This is further supported by the non-essentiality of NSUN2 in normal mouse model [47] . 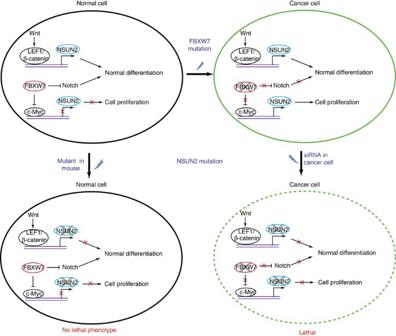Figure 5: A cancer drug target revealed by predicted negative genetic interactions. NSUN2is predicted to have a negative genetic interaction withFBXW7. TargetingNSUN2can kill the cancer cells while leaving the normal cell relatively unaffected. In normal cells, the tumour-suppressor geneFBXW7has functional redundancy withNSUN2in regulating cellular differentiation. In cancer cells, loss of function ofFBXW7results in an elevated expression of c-Myc. Activation of c-Myc results in the upregulation of NSUN2 that is essential for cell proliferation. Owing to a synthetic lethality betweenFBXW7andNSUN2, targetingNSUN2kills cancer cells, while leaving normal cells relatively unaffacted. A solid line represents an active protein, for example, FBXW7 inhibiting the accumulation of NOTCH1 and NOTCH3 in normals cells45. A red cross illustrates the disruption of the function of a protein, that is, transcriptional regulation ofNSUN2by c-Myc2 is repressed in normal cell, or the disruption of a cellular function, that is, differentiation or proliferation. Figure 5: A cancer drug target revealed by predicted negative genetic interactions. NSUN2 is predicted to have a negative genetic interaction with FBXW7 . Targeting NSUN2 can kill the cancer cells while leaving the normal cell relatively unaffected. In normal cells, the tumour-suppressor gene FBXW7 has functional redundancy with NSUN2 in regulating cellular differentiation. In cancer cells, loss of function of FBXW7 results in an elevated expression of c-Myc. Activation of c-Myc results in the upregulation of NSUN2 that is essential for cell proliferation. Owing to a synthetic lethality between FBXW7 and NSUN2 , targeting NSUN2 kills cancer cells, while leaving normal cells relatively unaffacted. A solid line represents an active protein, for example, FBXW7 inhibiting the accumulation of NOTCH1 and NOTCH3 in normals cells [45] . A red cross illustrates the disruption of the function of a protein, that is, transcriptional regulation of NSUN2 by c-Myc2 is repressed in normal cell, or the disruption of a cellular function, that is, differentiation or proliferation. Full size image Even though various experimental techniques are available to study protein function, understanding their functions within protein complexes and their relationships between each other in a complex remains a challenge. Here, we have developed a model to predict functional relationships within protein complexes using the evolutionary history of genomes in terms of gene gain and loss events. We first focused on the relationships in which the function of one protein A depends on the function of another protein B, but in which the reverse relationship is much weaker. We predicted such asymmetry by integrating various evolutionary scenarios, such as, gene B is more frequently gained across evolutionary history in the absence of gene A than vice versa . So, B can occur without A, but A cannot occur without B. To validate the method, we showed that the predicted functional asymmetry is consistent with various sources of empirical evidence, such as asymmetry in gene essentiality and single-knockout growth defects. However, one-third of the gene pairs in the same complex with asymmetry in gene essentiality (633/2,130) have not been captured by our model. Perfect prediction can, however, not be expected, because it is strictly based on complete gene loss and gain. Our model may therefore benefit from more fine-scale evolutionary events, such as the incorporation of mutation rates. Thus, in species where both A and B are still present, there might be asymmetry in the extent to which they have diverged at the sequence level from their respective ancestors. Second, the essentiality and growth defect data sets [4] , [49] cover specific nutrient environments, which might not be experienced by species in our evolutionary model. Such differences in physiological conditions may result in different genome evolution and, as such, it could negatively affect model predictions. Interestingly, functional asymmetric relationships can be used to predict negative genetic interactions in those cases where multiple proteins, for instance, A and C, have asymmetry with the same protein B. The underlying idea is that functional asymmetry is owing to the fact that A and C can compensate for each other’s absence. Indeed, we have shown that our model increases the predictive power for negative genetic interactions in S. cerevisiae protein complexes by 50–100% relative to random protein pairs from the same complex. Moreover, we predict many novel genetic interactions, of which eight have been experimentally verified in S. pombe and D. melanogaster . Although this number is not high, this is not unexpected given that genome-scale genetic interaction screens have only been performed in S. cerevisiae [20] and S. pombe [50] . Moreover, only one screen under standard nutrient condition has been conducted for these two species, respectively, and it remains to be seen how genetic interactions vary across other nutrient conditions. It would therefore be interesting to apply our model to study the variation of interactions across conditions, for example, to re-evaluate evolutionary theories that are based on adaptive landscapes (for example, robustness against mutations in single environments) initialized by studies on metabolism [51] . One strategy would be to integrate gene expression profiles across a wide range of nutrient conditions with protein complex data to remove unexpressed subunits from protein complexes and thus obtain condition-specific complexes. In addition, condition-specific essentiality profiles [4] could be used to constrain the independent protein (B) to be essential. As a result, one could predict fan-in motifs that are specific for a given condition. Our finding that the predictive power of negative genetic interactions doubles when incorporating essentiality supports such a strategy. Various recent studies have stated that the discovery of (negative) genetic interactions is a very important step towards a full understanding of the genetic basis of complex diseases and providing a framework to discover drug targets [52] , [53] , [54] . Even though there are a number of very promising candidate drug targets discovered by using genetic interactions [10] , [11] , effectively identifying them experimentally remains a major challenge. In contrast to other prediction models [12] , [13] , [18] , our model does not depend on genetic interaction screens, which are available in a very limited number of species. Thus, our model can be applied to predict genetic interactions in species even when no empirical genetic interaction information is available. Moreover, compared with Pandey et al. [18] , our model has a significantly higher prediction precision. Our approach is therefore useful to prioritize drug candidates. We found 20 cancer drug targets for which there is empirical evidence that they are essential in tumour cells and predicted ten novel drug targets. Notably, the majority (25/30) has not been measured in yeast or predicted by other computational approaches [13] , [18] . These targets are promising given the empirical evidence that all are essential in at least one cancer type, such as breast, pancreas or ovarian cancer, while non-essential in model organisms. Future studies should reveal to what extent these targets are (i) non-essential in the same human healthy cell type, (ii) conserved across different tumour types and (iii) vulnerable for drug compounds. In the light of medical genetics, the presented approach can be applied to mammals when future protein–protein interaction networks become available for cancer and normal cell lines. This would allow for more specific predictions of cancer drug targets. It should be noted that although we focused on protein complexes, our model might be used to predict interactions for any gene pair, as long as they are known to have a functional relationship between them. Taken together, this study shows that negative genetic interactions in protein complexes can be predicted by genome evolution, which has an application in searching for drug targets and in understanding human diseases. Protein complexes Four hundred and nine and 2,468 protein complexes of S. cerevisiae [17] and human [34] , [35] were used to predict negative genetic interactions within them, respectively. For each protein complex, all pair-wise combinations of proteins were generated as input for our evolutionary model. Reconstruction of ancestral states We used the presence and absence of orthologous genes across 373 species obtained from STRING 7.0 orthologous groups [29] to reconstruct ancestral states of genes. We inferred the most parsimonious ancestral presence/absence states of each gene by using a rooted trifurcation (Achaea/Eukaryote/Eubacteria) phylogenetic tree of 373 species. All results were obtained using a gain/loss cost ratio of 2/1 and a delayed transition assumption (DELTRAN) in PAUP [55] . From the ancestral state reconstruction, we generated 11 evolutionary variables as inputs to the following classification step. The integration of these 11 evolutionary variables gives the highest correct classification rate compared with alternative integrations of evolutionary variables. For each gene pair A–B, we examined the following six evolutionary scenarios: (i) both genes were absent in the ancestor (a) and one was gained in the descendant (d) (a00_d10 or a00_d01), (ii) the presence of only one gene in the ancestor was maintained in the descendant (a10_d10 or a01_d01), (iii) both genes were present in the ancestor and one was lost in the descendant (a11_d01 or a11_d10), (iv) a gain of one gene occurred when the other was present in the ancestor (a01_d11 or a10_d11), (v) only one gene was present in the ancestor and was lost in the descendant (a10_d00 or a01_d00) and (vi) only one gene was present in the ancestor and was lost in the descendant while the other gene was gained (a10_d01 or a01_d10) ( Fig. 2b ). For gene A, we also calculated five fractions that reflect evolutionary asymmetry between A and B, f 1 : a11_d01/(a11_d01+a11_d10), f 2 : a01_d11/(a01_d11+a10_d11), f 3 : a01_d01/(a01_01+a10_d10), f 4 : a01_d11/(a01_d11+a00_d10) and f 5 : a01_d11*[a01_d11−a00_d10+1]/[a01_d11+a00_d10]. Evolutionary information to predict asymmetry of gene pairs First, we reconstructed ancestral states for 2,400 directionally coupled enzyme pairs (functional asymmetry; A→B) in the yeast metabolic network [19] and generated the 11 evolutionary variables. Directional coupling was found by constraining the reaction flux of one to a finite value followed by minimizing and maximizing another, and vice versa [14] . A→B is found when the minimum flux through A is zero while the maximum is a finite value (when constraining B to a finite flux), and the minimum and maximum flux through B is unequal to zero when A is constrained to a finite value. Thus, the activity of A depends on the activity of B, but not the reverse (A→B). Each of the 11 evolutionary variables is a predictor for functional asymmetry between an enzyme pair (A→B) as the 11 variables of a dependent A differ from those of an independent B. More specifically, for evolutionary events (i) and (ii), A is expected to occur less often than the independent B. For the other four evolutionary events, A is expected to occur more often than the independent B. Furthermore, we expect f 1 , f 2 , f 3 and f 4 to be larger than 0.5, and f 5 to be larger than 0 for asymmetric functional relationships ( Supplementary Fig. S1 ). Given the fact that these 11 variables are not independent from each other, we used a Tree Augmented Naïve Bayes (TAN) classifier to integrate these predictors. The TAN classifier relaxes the assumption of independence of input variables. The classifier is trained on the 2,400 directionally coupled enzyme pairs using WEKA [56] . The classifier estimates conditional probabilities of one gene being independent ( α 1 ) or dependent ( α 2 ), where α 1 + α 2 =1. The gene is predicted to be either independent (if α 1 > α 2 ) or dependent (if α 1 < α 2 ) with a conditional probability ( α ), where α =max ( α 1 , α 2 ). To predict the functional relationship in protein complexes by this classifier, we first reconstructed ancestral states for 8,711 protein pairs (A–B) and generated the 11 evolutionary variables for A and B. The functional relationship of A–B is determined as follows: (i) the classifier generates class predictions for A with a probability estimate ( α ); (ii) identifying predictions with high confidence by a cutoff on α (any prediction where α is smaller than the cutoff remains unclassified); (iii) protein B is predicted in the same way; and (iv) combining the classification result of A and B, A–B is predicted as functionally asymmetric when A is dependent and B is independent or vice versa . Otherwise, there is no evidence for functional asymmetry and the pair becomes unclassified ( Fig. 2c ). Gene essentiality Essentiality data were obtained from MIPS database [49] . If a gene is annotated as both essential and non-essential in different sources, the essentiality is assigned according to the majority rule. Otherwise, a gene was marked as ambiguous. For predicted asymmetric pairs (A→B), we counted cases where only B is essential ( n 01 ) and cases where only A is essential ( n 10 ). For symmetric pairs (A–B), it is expected that n 01 is equal to n 10 . To test against the null hypothesis of no relationship between predicted functional asymmetry and asymmetry in essentiality, we subjected the 2 × 2 contingency table of essential/non-essential versus symmetric/asymmetric to a one-tailed Fisher’s exact test. Growth defect of single-gene knockouts in rich medium Growth defect of single-gene knockouts was obtained from two studies [20] , [21] , which cover 75% of all genes in S. cerevisiae . A growth defect was considered as substantial if a gene knockout causes a growth defect >10% (ref. 4 ). For predicted asymmetric pairs with two non-essential genes (A→B), we counted cases where knockout of B causes a more severe growth defect ( n 01 ) and cases where knockout of A causes a more severe growth defect ( n 10 ). For functional symmetric pairs (A–B), it is expected that n 01 is equal to n 10 . To test against the null hypothesis of no relationship between predicted functional asymmetry and asymmetry in growth defect, we subjected the 2 × 2 contingency table of n 01 / n 10 versus symmetric/asymmetric to a one-tailed Fisher’s exact test. Negative genetic interactions in the metabolic network We obtained fan-in motif A–C pairs for metabolic reactions ( Fig. 1c ) by using flux coupling between enzymes within the genome-scale metabolic network of S. cerevisiae (see above). The fan-in motif A–C pairs have two characteristics: (i) A and C both depend on a third essential protein B (A→B and C→B) and (ii) the A–C pair is uncoupled. For experimental validation, we used an empirical genetic interaction profile from Szappanos et al. (obtained from the Supplementary Information [21] ). If no significant genetic information was available for a pair of genes, we determined it as not measured and excluded it from the analysis. To test against the null hypothesis of no enrichment of negative genetic interactions in fan-in motif A–C pairs, we summarized the motif A–C/non-motif A–C pairs versus with/without negative genetic interaction in a 2 × 2 contingency table and subjected it to a one-tailed Fisher’s exact test. Negative genetic interactions in protein complexes We obtained A–C pairs with evolutionary fan-in motifs ( Fig. 1a ) from asymmetric functional relationships predicted by the TAN model ( Fig. 2c ). The evolutionary fan-in motif is characterized by (i) A and C depend on B, but not vice versa and (ii) A does not depend on C and vice versa . To ensure A–C is not an asymmetric pair, we applied the cutoff for significant functional asymmetry to α >=0.7. At this cutoff, the correct classification rate increases the most at the smallest cost of samples size ( Supplementary Fig. S4 ). Genetic interaction data were obtained from BioGRID [31] . As BioGRID does not specify whether the genetic interaction of a gene pair has been measured, we integrated the original data from nine high-throughput data sets [20] , [21] , [22] , [23] , [24] , [25] , [26] , [27] , [28] , to generate a list of measured genetic interactions (either positive, negative or no interaction). If a pair of genes has both a negative and a positive genetic interaction, the genetic interaction was assigned according to the majority rule. To test against the null hypothesis of no enrichment of negative genetic interactions in pairs with a fan-in motif, we summarized motif A–C/non-motif A–C versus with/without negative genetic interaction in a 2 × 2 contingency table and tested using a one-tailed Fisher’s exact test. Prediction of cancer drug targets We mapped predicted negative genetic interactions from yeast to human via orthology from STRING7.0 (ref. 29 ). To retrieve drug targets, we first mapped cancer gene information from the Cancer Genome Project [36] to the predicted genetic interactions to extract predictions involving one oncogene or tumour-suppressor gene. Then we mapped gene essentiality measurements in cancer from Marcotte et al. [38] to the predictions. In addition, non-essentiality of the drug targets in normal cells/tissues was examined by literature mining covering M. Musculus , D. melanogaster or D. rerio . To predict targets directly from human protein complexes, we trained our model on functional asymmetric enzyme pairs from the human genome-scale metabolic network [37] via Flux Coupling Analysis (see also above for yeast and Burgard et al. [14] ). Subsequently, we used experimentally determined protein complexes [34] , [35] to predict human-specific negative genetic interactions via the evolutionary fan-in motifs. Finally, we examined gene essentiality among predicted drug targets in cancer and normal cells/tissues as outlined above. How to cite this article: Lu, X. et al. Genome evolution predicts genetic interactions in protein complexes and reveals cancer drug targets. Nat. Commun. 4:2124 doi: 10.1038/ncomms3124 (2013).